Orthogonal ring-closing alkyne and olefin metathesis for the synthesis of small GTPase-targeting bicyclic peptides Bicyclic peptides are promising scaffolds for the development of inhibitors of biological targets that proved intractable by typical small molecules. So far, access to bioactive bicyclic peptide architectures is limited due to a lack of appropriate orthogonal ring-closing reactions. Here, we report chemically orthogonal ring-closing olefin (RCM) and alkyne metathesis (RCAM), which enable an efficient chemo- and regioselective synthesis of complex bicyclic peptide scaffolds with variable macrocycle geometries. We also demonstrate that the formed alkyne macrocycle can be functionalized subsequently. The orthogonal RCM/RCAM system was successfully used to evolve a monocyclic peptide inhibitor of the small GTPase Rab8 into a bicyclic ligand. This modified peptide shows the highest affinity for an activated Rab GTPase that has been reported so far. The RCM/RCAM-based formation of bicyclic peptides provides novel opportunities for the design of bioactive scaffolds suitable for the modulation of challenging protein targets. Macrocyclic peptides exhibit unique surface recognition properties and allow the stabilization of bioactive peptide conformations resulting in ligands with increased bioactivity and bioavailability [1] , [2] , [3] , [4] , [5] . Such scaffolds already proved useful for the modulation of biological targets which are intractable by typical small molecules, such as transcription factors and small GTPases [6] , [7] , [8] , [9] , [10] , [11] , [12] . Recently, structurally rigid bicyclic peptides obtained mainly by epitope grafting on disulfide-rich frameworks [13] , [14] or by phage-display screening [15] , [16] have emerged as particularly interesting inhibitor types. Given the potential of this new chemical modality as scaffold for next-generation therapeutics, the development of efficient synthetic methods that enable the introduction of non-natural fragments into peptidic bicycles is in high demand. This is particularly true for approaches that allow the design of scaffolds that go beyond the size of small epitopes. For the synthesis of monocyclic peptides, a variety of methods is available [17] , [18] , [19] , [20] , [21] , [22] , [23] , [24] , [25] . Notably, in such peptides, the crosslink itself can directly contribute to bioactivity [26] , [27] , [28] . In this respect, hydrocarbon crosslinks formed by ruthenium-catalysed ring-closing olefin metathesis (RCM) proved particularly successful owing to the hydrophobic and inert character of those crosslinks [2] , [29] . Prominent examples involve hydrogen bond surrogates [8] , [30] , [31] and hydrocarbon stapling [32] , [33] , [34] , [35] , which have provided a number of potent inhibitors of protein—protein interactions [2] . In these cases, the synthesis of bicyclic architectures requires the presence of multiple olefins, which causes selectivity problems during cyclization [36] , [37] . Undesired side reactions can be reduced by the selection of appropriate ring sizes and distances [38] , by functional group transformations [39] and by tedious fine tuning of olefin reactivity [39] . Thus, only a small set of scaffolds is accessible by multiple RCM reactions [36] , [37] , [38] , [39] , [40] . This creates the need for synthesis methods that integrate two consecutive, chemically orthogonal metathesis reactions thereby enabling efficient chemo- and regioselective construction of complex bicyclic peptides. Ideally, such methods would be compatible with solid-phase peptide synthesis (SPPS). Molybdenum-catalysed ring-closing alkyne metathesis [41] (RCAM) shares many of the advantageous properties of RCM, and is in principle chemically orthogonal to ruthenium-catalysed RCM. RCAM has been applied for peptide macrocyclizations in solution [42] , [43] , [44] . However, the synthesis of bicyclic peptides by orthogonal ring-closing olefin and alkyne metathesis has not been explored so far. Here, we report the solid-phase synthesis of bicyclic peptides by means of orthogonal ring-closing olefin- and alkyne-metathesis reactions. We demonstrate that the alkyne macrocycle can be further functionalized selectively. The orthogonal RCM/RCAM system was successfully used to evolve a monocyclic peptide inhibitor of the small GTPase Rab8 into a bicyclic ligand with increased target affinity. RCAM and functionalization on solid support To explore RCAM-based macrocyclization of peptides on solid support ( Fig. 1a ), two α-methyl-α-alkynyl building blocks ( 1 – 4 ) of varying linker length and configuration ( Fig. 1b ) were introduced into model peptides using Fmoc-based SPPS. Peptide sequences, architectures and relative spacing of non-natural amino acids ( i , i +3, i , i +4 and i , i +7) were selected by analogy to previously explored RCM-based peptide macrocyclizations [33] . As proof-of-concept and to test the robustness of the reaction, we designed model peptides that contain all functionalities present among the 20 proteinogenic amino acids and yield macrocyclic peptides 7 – 9 after RCAM ( Fig. 2a ). 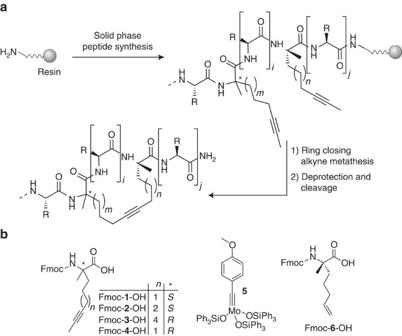Figure 1: Alkyne macrocyclization. (a) The linear peptide is assembled via SPPS including the incorporation of two α-methylated-α-alkynylated building blocks (1–4). The C-terminal building block is always (S)-configured, the configuration of the N-terminal building block varies between the different architectures. Complex5is used to perform the RCAM reaction. (i=2, 3, 6, number of amino acids between non-natural building blocks;j=3, 6;m=1, 2, 4;n=1, 2; R=side chain of a proteinogenic amino acid) (b) Fluorenylmethoxycarbonyl (Fmoc) protected non-natural amino acids incorporated into the peptide sequence (alkyne:1–4, olefin:6). The alkyne building blocks1–4are either used in the (S)- or (R)-configuration depending on the macrocycle architecture. Mo-complex (5) used for RCAM. Investigation of various RCAM conditions including the latest generation of stable Mo-complexes [45] , [46] ( Supplementary Table 1 ) revealed efficient conversions after 3 h at 40 °C in toluene if Tentagel rink amide resin and complex 5 ( Fig. 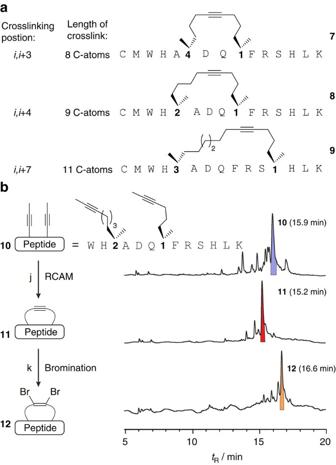Figure 2: Ring-closing alkyne metathesis on solid support. (a) Sequences of peptides7–9containing different macrocylic architectures. (b) Sequence of peptide10with non-natural amino acids1and2at positioniandi+4 (nine-carbon crosslink) with corresponding chromatograms of crude reaction mixtures before (10, top) and after RCAM (11, middle) and after dibromination (12, bottom). Corresponding product peaks are highlighted: open (10, blue), closed (11, red) and dibrominated (12, orange) macrocycle. Chromatograms were obtained after deprotection and release of intermediates from the resin. ‘j’ represents Complex5, dry toluene, 40 °C, 2 × 1.5 h; ‘k’ represents CuBr2, dry MeCN, 3 × 1 h. 1a ) were used ( Supplementary Figs 2–5 , Supplementary Table 2 ). Under these conditions, macrocycles were formed for all three architectures ( 7 – 9 ) with the best results obtained for an i , i +4 geometry and a final crosslink of nine carbon atoms ( 8 ). Shortening the hydrocarbon bridge from nine to eight carbon atoms reduces the efficiency of the reaction presumably due to increased ring strain ( Supplementary Fig. 4 ). Figure 1: Alkyne macrocyclization. ( a ) The linear peptide is assembled via SPPS including the incorporation of two α-methylated-α-alkynylated building blocks ( 1 – 4 ). The C-terminal building block is always ( S )-configured, the configuration of the N-terminal building block varies between the different architectures. Complex 5 is used to perform the RCAM reaction. ( i =2, 3, 6, number of amino acids between non-natural building blocks; j =3, 6; m =1, 2, 4; n =1, 2; R=side chain of a proteinogenic amino acid) ( b ) Fluorenylmethoxycarbonyl (Fmoc) protected non-natural amino acids incorporated into the peptide sequence (alkyne: 1 – 4 , olefin: 6 ). The alkyne building blocks 1 – 4 are either used in the ( S )- or ( R )-configuration depending on the macrocycle architecture. Mo-complex ( 5 ) used for RCAM. Full size image Figure 2: Ring-closing alkyne metathesis on solid support. ( a ) Sequences of peptides 7 – 9 containing different macrocylic architectures. ( b ) Sequence of peptide 10 with non-natural amino acids 1 and 2 at position i and i +4 (nine-carbon crosslink) with corresponding chromatograms of crude reaction mixtures before ( 10 , top) and after RCAM ( 11 , middle) and after dibromination ( 12 , bottom). Corresponding product peaks are highlighted: open ( 10 , blue), closed ( 11 , red) and dibrominated ( 12 , orange) macrocycle. Chromatograms were obtained after deprotection and release of intermediates from the resin. ‘j’ represents Complex 5 , dry toluene, 40 °C, 2 × 1.5 h; ‘k’ represents CuBr 2 , dry MeCN, 3 × 1 h. Full size image Selective functionalization of the alkyne linker embedded in the macrocycle was achieved, after treatment of macrocyclic peptide 11 with CuBr 2 in dry acetonitrile on solid support to yield dibrominated olefin 12 ( Fig. 2b ). Notably, the reaction can be performed conveniently with different resin-bound peptides (for all tested architectures: i , i +3, i , i +4 and i , i +7) using standard syringe reactors ( Supplementary Figs 6–8 , Supplementary Table 2 ). Full conversion in the dibromination reaction is only achieved after multiple treatments with CuBr 2 and for peptides that lack the two N-terminal sulfur containing amino acids (Cys and Met). Bicyclic peptide synthesis via orthogonal RCM and RCAM To determine whether RCM and RCAM can be performed orthogonally within one peptide sequence ( Fig. 3a ), peptide 16 was synthesized which embodies two alkyne-functionalized building blocks ( 1 and 2 ) in i , i +4-position at the carboxy (C) terminus, and two olefin-containing amino acids ( 6 , Fig. 1b ) in i , i +4-position at the amino (N) terminus ( Fig. 3b ). In peptide 16 , an olefin macrocycle can be formed next to an alkyne-bearing macrocycle ( Fig. 3b ). The treatment of immobilized precursor peptide 13 (blue peak) with either complex 5 or Grubbs first-generation catalyst leads to selective formation of the alkyne ( 14 , red peak) and olefin macrocycle ( 15 , orange peak), respectively ( Fig. 3b , Supplementary Figs 9 and 10 ). HPLC-MS analyses of the alkyne and olefin crosslinked intermediates ( 14 and 15 ) reveal highly selective formation of the desired macrocycle without formation of an alternative cyclization product ( Supplementary Fig. 10 ). Both monocycles can be converted into the bicyclic product 16 by means of the second metathesis reaction. This result is remarkable since previous attempts of orthogonal macrocycle formation within peptides failed [44] , but were successful only for the assembly of simple building blocks [47] . In an even more demanding set-up, the simultaneous closure of both macrocycles in a one-pot reaction was tested (instead of the previous sequential synthesis). Strikingly, treatment of the open peptide precursor 13 with a mixture of complex 5 and Grubbs first-generation catalyst also yields the desired bicyclic peptide 16 (green peak, Fig. 3b and Supplementary Fig. 10 ). 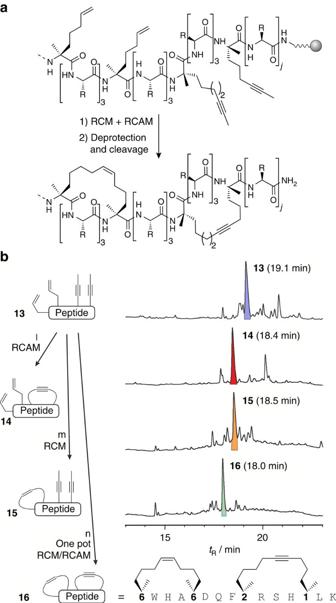Figure 3: Solid phase synthesis of bicyclic peptides by means of the RCM/RCAM method. (a) General scheme for the synthesis of bicyclic peptides obtained by means of RCM and RCAM of the acyclic precursor peptides. (j=2, number of C-terminal amino acids; R=side chain of a proteinogenic amino acid except Cys or Met). (b) Sequence of bicyclic test peptide16bearing ani,i+4 olefin crosslink (eight C-atoms) and ani,i+4 alkyne crosslink (nine C-atoms). Chromatograms of crude reaction mixtures of peptide16before macrocyclization (13, top), after RCAM (14, second) and RCM (15, third), respectively, and after simultaneous (one-pot) RCM and RCAM (16, bottom). Corresponding product peaks are highlighted: fully open (13, blue), alkyne monocycle (14, red), olefin monocycle (15, orange) and bicyclic peptide (16, green). Chromatograms were obtained after deprotection and cleavage of resin-bound intermediates. ‘l’ represents Complex5, dry toluene, 40 °C, 2 × 1.5 h; ‘m’ represents Grubbs first-generation catalyst, DCE, 3 × 2 h; ‘n’ represents Complex5, Grubbs first-generation catalyst, dry toluene, 40 °C, 2 × 1.5 h. Figure 3: Solid phase synthesis of bicyclic peptides by means of the RCM/RCAM method. ( a ) General scheme for the synthesis of bicyclic peptides obtained by means of RCM and RCAM of the acyclic precursor peptides. ( j =2, number of C-terminal amino acids; R=side chain of a proteinogenic amino acid except Cys or Met). ( b ) Sequence of bicyclic test peptide 16 bearing an i , i +4 olefin crosslink (eight C-atoms) and an i , i +4 alkyne crosslink (nine C-atoms). Chromatograms of crude reaction mixtures of peptide 16 before macrocyclization ( 13 , top), after RCAM ( 14 , second) and RCM ( 15 , third), respectively, and after simultaneous (one-pot) RCM and RCAM ( 16 , bottom). Corresponding product peaks are highlighted: fully open ( 13 , blue), alkyne monocycle ( 14 , red), olefin monocycle ( 15 , orange) and bicyclic peptide ( 16 , green). Chromatograms were obtained after deprotection and cleavage of resin-bound intermediates. ‘l’ represents Complex 5 , dry toluene, 40 °C, 2 × 1.5 h; ‘m’ represents Grubbs first-generation catalyst, DCE, 3 × 2 h; ‘n’ represents Complex 5 , Grubbs first-generation catalyst, dry toluene, 40 °C, 2 × 1.5 h. Full size image In peptide 16 , the two individual macrocycles are sequentially arranged along the amino acid chain, that is, the two individual macrocycles are linked by a linear amino acid sequence. A synthetically more challenging setup involves the synthesis of two entangled macrocyles resulting in more constrained peptide scaffolds (for example, peptide 17 , Fig. 4 ). In this architecture, an edge-on bimacrocycle structure is generated as opposed to a linear macrocycle arrangement as in peptide 16 . Most notably, entangled bicyclic peptide 17 ( Fig. 4 ) was also efficiently formed in both the sequential as well as the one-pot synthesis ( Supplementary Figs 11 and 12 ). 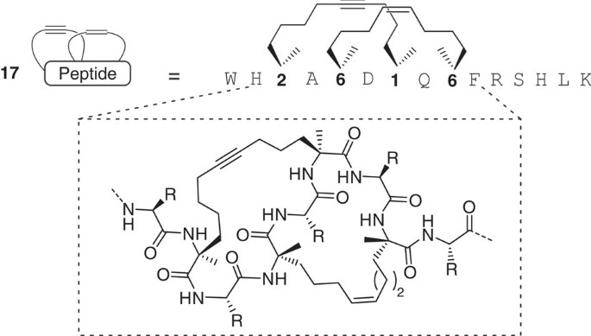Figure 4: Sequence and chemical structure of the engulfed bicyclic peptide 17. R, side chain of a proteinogenic amino acid except Cys or Met. Figure 4: Sequence and chemical structure of the engulfed bicyclic peptide 17. R, side chain of a proteinogenic amino acid except Cys or Met. Full size image Bicyclic ligands of the small GTPase Rab8 To demonstrate the potential of this robust orthogonal RCM/RCAM macrocyclization, we aimed at the improvement of a monocyclic bioactive peptide targeting a challenging protein. Small GTPases comprise a protein superfamily with clinically highly relevant, yet particularly challenging, drug targets [48] , [49] , [50] , [51] , [52] , [53] , [54] . Despite enormous efforts, no efficient inhibitors of small GTPases have reached clinical trials. Importantly, the target affinity of small molecule modulators typically does not exceed the low-to-medium micromolar range [50] , [51] . Among the small GTPase superfamily, Rab proteins (Ras-related in brain) constitute key regulators of intracellular vesicular transport and trafficking [55] , [56] . As starting point for the generation of a bicyclic peptide, we selected the hydrocarbon-stapled monocyclic peptide StRIP3 , which binds the small GTPase Rab8a with moderate affinity (dissociation constant ( K d )=20.7 μM, Table 1 , entry 2) [12] . StRIP3 resembles the only known inhibitor of a Rab protein–protein interaction [12] and is based on the interaction motif of Rab6-interacting protein 1 ( wt-R6IP , Table 1 , entry 1) [57] . Initially, alkyne-bearing macrocycles based on StRIP3 were explored in which the i , i +4 olefin crosslink was replaced by alkynes with varying crosslink length (9–10 carbon atoms, Table 1 , entry 3–5). The 10-carbon crosslink requires double incorporation of building block 2 (entry 3). A nine-carbon crosslink is generated by incorporation of two different building blocks ( 1 and 2 ), which results in two different architectures (entry 4: 1 / 2 , entry 5: 2 / 1 ). The synthesis of an eight-carbon crosslinked StRIP3 derivative containing building block 1 twice was not possible, most likely due to high ring strain caused by the linear geometry of the triple bond. Table 1 Small GTPase targeting peptides. Full size table In addition, dibrominated (entry 6–8) and bicyclic peptides (entry 9–14) were synthesized resulting in a total of 12 StRIP3 derivatives grouped into four subfamilies ( Table 1 , Supplementary Table 3 ): (i) alkyne mono-macrocyclic peptides 18 – 20 (entry 3–5); (ii) dibrominated olefin macrocyclic peptides 21 – 23 (entry 6–8); (iii) orthogonally macrocyclized peptides 24 – 26 carrying the original olefin crosslink and an additional alkyne crosslink at the C terminus (entry 9–11); and (iv) bicyclic peptides 27 – 29 with exchanged positions for the alkyne and the olefin crosslink (entry 12–14). Since the N-terminal part of parent peptide StRIP3 is already constrained by the olefin macrocycle, we aimed for the introduction of a new macrocycle in the C-terminal part. We reasoned that additional constraint could further stabilize the bioactive peptide conformation. Owing to a lack of structural information, it is not obvious which amino acids are directly involved in Rab-binding. For this reason, we selected two amino acids with hydrophobic side chains (L911 and A915) for macrocycle introduction as their non-polar side chains are potentially mimicked by the hydrocarbon macrocycle. All the peptides were synthesized via SPPS and modified with an N-terminal fluorescein–polyethyleneglycol label ( Supplementary Table 3 ) to enable determination of their binding affinity towards activated Rab8a 6-176 (GppNHp) in a fluorescence polarization (FP) assay ( Supplementary Fig. 13 ). After initial ranking of the peptides by means of relative K d values (rel. K d , Table 1 , Supplementary Table 4 ), the affinity of the best binders (peptide 21 , 25 and 28 ) was determined in an independent FP assay run in triplicates ( Table 1 , Supplementary Fig. 14 ). Replacement of the olefin by an alkyne crosslink yields peptides 18 – 20 with affinities comparable to StRIP3 . In contrast, the dibrominated olefin derivatives 21 – 23 show improved affinity towards Rab8a 6–176 with peptide 21 being the most potent binder within this subfamily ( K d =10.7 μM, Table 1 ). Peptide 21 shows a 2-fold increased binding affinity when compared with StRIP3 . Notably, an even higher improvement in binding affinity to Rab8a 6–176 (GppNHp) is observed for two of the bicyclic peptides 24 – 29 , namely peptide 25 and 28 ( Table 1 and Supplementary Table 4 ). In both the cases, the nine-carbon alkyne crosslink (with 1 at N-terminal and 2 at C-terminal position within the sequence) provides the most potent architecture resulting in two significantly improved ligands for activated Rab8a 6–176 ( K d [ 25 ]=6.6 μM; K d [ 28 ]=9.6 μM). Bicyclic peptide 25 ( Fig. 5a ) is more than three times more potent than the parent hydrocarbon stapled peptide StRIP3 and displays a more than 15-fold increased binding affinity compared with the unmodified wild-type peptide wt-R6IP . Binding affinity of peptide 25 was confirmed in microscale thermophoresis measurements. 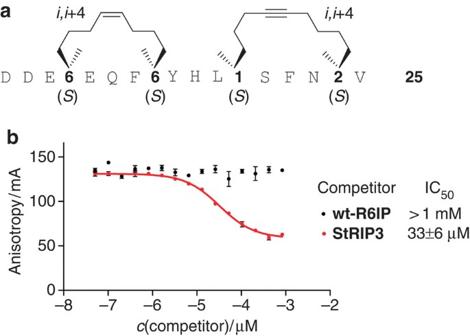Figure 5: Sequence and binding studies of peptide 25. (a) Sequence of bicyclic peptide25showing highest affinity for Rab8a6–176(GppNHp). (b) Competition of fluorescein-labelled peptide25(60 nM) bound to Rab8a(GppNHp; 15 μM) with increasing concentrations of acetylated peptidesStRIP3andwt-R6IP(competitors). Errors represent 1σ of triplicates. On the basis of fluorescence intensity, an affinity for Rab8a 6–176 (GppNHp) was observed ( K d [ 25 ]=11 μM, Supplementary Table 5 , Supplementary Figs 15 and 16 ), which is in the range of our FP measurements ( K d [ 25 ]=6.6 μM, see above). In addition, FP competition experiments were performed using a complex between labelled peptide 25 and Rab8a 6–176 (GppNHp), which was treated with an excess of acetylated StRIP3 . In this setup, we observed full displacement of peptide 25 (IC 50 =33 μM, red Fig. 5b ). As one would expect, the acetylated low-affinity peptide wt-R6IP does not compete with peptide 25 (black, Fig. 5b ). These results verify reversible binding of peptide 25 to the same site on Rab8 as parent peptide StRIP3 . Figure 5: Sequence and binding studies of peptide 25. ( a ) Sequence of bicyclic peptide 25 showing highest affinity for Rab8a 6–176 (GppNHp). ( b ) Competition of fluorescein-labelled peptide 25 (60 nM) bound to Rab8a(GppNHp; 15 μM) with increasing concentrations of acetylated peptides StRIP3 and wt-R6IP (competitors). Errors represent 1σ of triplicates. Full size image We identified conditions that enable the performance of RCAM reactions in conjunction with SPPS allowing alkyne-based macrocyclization of peptide sequences involving all natural side-chain functionalities. Subsequent functionalization of the alkyne allows further modification of the macrocycle, which opens new perspectives in the design of macrocyclic scaffolds. In addition, we report the chemo- and regioselective synthesis of bicyclic peptides bearing an alkyne as well as an olefin crosslink accessible via orthogonal ring-closing olefin and alkyne metathesis on solid support. This approach allows direct control of the individual macrocyclization reaction and enables the formation of bicyclic peptides with novel architectures combining two different macrocycles within the same peptide sequence. The applicability of such scaffolds for highly challenging targets, such as small GTPases, was demonstrated via identification of the currently most potent binder of an activated Rab GTPase (peptide 25 , K d =6.6 μM). Since the bioactivity of a peptide is mainly determined by its secondary structure [1] , [2] , alkyne macrocyclization and the orthogonal introduction of bicyclic alkyne/olefin macrocycles within the same peptide sequence give rise to novel constrained peptide architectures with high potential for the targeting of currently intractable proteins. General For abbreviations and detailed information about the experimental procedures, analytical data and FP binding curves, see Supplementary Figs 1–16 , Supplementary Tables 1–5 , Supplementary Note 1 and Supplementary Methods . Synthesis of building blocks 1 – 4 Synthesis of the Fmoc protected building blocks 1 – 4 was performed according to adapted protocols using Ni(II)-BPB (( R/S )-2-[N-(N′-benzylpropyl)amino]benzophenone) complexes [58] , [59] . For a detailed description of building block synthesis and analytical data, see Supplementary Methods . Peptide synthesis Peptides were synthesized according to standard Fmoc-chemistry for SPPS using HCTU ( O -(6-chlorobenzotriazol-1-yl)- N , N , N ′, N ′-tetramethyluronium hexafluorophosphate) and COMU (1-[(1-(cyano-2-ethoxy-2-oxoethylidenaminooxy)-dimethylaminomorpholino)]-uronium hexafluorophosphate) as coupling reagents ( Supplementary Fig. 1 ). For more detailed information about peptide synthesis, see Supplementary Methods and Supplementary Tables 2 and 3 . Ring-closing alkyne metathesis The dried resin was swollen and shrunken under argon alternating in dry diethyl ether and dry toluene (3 × each). Afterwards 0.5 ml of a solution of the alkyne-metathesis complex 5 (2 mg ml −1 ) in dry toluene was added and the reaction mixture was stirred at 40 °C for 1.5 h. During the reaction time, argon was bubbled through the reaction mixture to evaporate the 2-butyne. After addition of 0.5 ml of fresh complex 5 solution, the mixture was stirred at 40 °C for 1.5 h. Ring-closing olefin metathesis The dried resin was swollen in 1,2-dichloroethane (DCE) for 15 min. Subsequently, 0.5 ml of a solution of Grubbs first-generation catalyst (2 mg ml −1 ) in DCE was added to the resin and reacted for 2 h at room temperature. During the reaction time, argon was bubbled through the reaction mixture to remove ethene. The procedure was repeated twice. One-pot ring-closing alkyne and olefin metathesis The dried resin was swollen and shrunken under argon alternating in dry diethyl ether and dry toluene (3 × each). Afterwards 0.5 ml of a solution of the alkyne-metathesis complex 5 (2 mg ml −1 ) and Grubbs first-generation catalyst (2 mg ml −1 ) in dry toluene was added and the reaction mixture stirred at 40 °C for 1.5 h. During the reaction time, argon was bubbled through the reaction mixture to evaporate 2-butyne and ethene. After the addition of 0.5 ml of fresh complex solution (alkyne complex 5 and Grubbs first-generation catalyst), the mixture was stirred at 40 °C for 1.5 h. Dibromination of alkyne macrocycles The dried resin was swollen in dry MeCN for 15 min and treated with a mixture of CuBr 2 in dry MeCN (2 mg ml −1 ) for 2 h. The reaction was performed in a Syringe reactor and the procedure was repeated twice. Protein expression and purification The expression and purification of Rab8a 6–176 was performed by analogy to full-length Rab8a according to established protocols [60] , [61] . Nucleotide exchange Nucleotide exchange was performed according to previously established protocols [60] , [62] . Briefly, for nucleotide removal, Mg 2+ was removed by the addition of a 5-fold excess of EDTA and reacted for 1 h at room temperature. The protein solution was desalted using a PD-10 desalting column Sephadex G-25 DNA Grade (GE Healthcare) with elution buffer consisting of 20 mM HEPES (pH 7.5), 50 mM NaCl, 1 mM TCEP. After removal of Mg 2+ , the protein was diluted to 80–100 μM before the addition of ZnCl 2 (500 μM) and (NH 4 ) 2 SO 4 (200 mM). After the addition of alkaline phosphatase (5 U mg −1 Rab protein), the mixture was incubated for 16 h at 4 °C. For nucleotide exchange, the mixture contained a 5-fold excess of GppNHp during alkaline phosphatase incubation. Afterwards, the mixture was desalted using a PD-10 desalting column Sephadex G-25 DNA Grade (GE Healthcare) with elution buffer consisting of 25 mM HEPES (pH 7.5) 150 mM NaCl, 1 mM TCEP, 1 mM MgCl 2 and 1 μM GppNHp. Fluorescence polarization assay Rab8a 6–176 (GppNHp) was serially diluted in a buffer containing 25 mM HEPES (pH 7.5), 150 mM NaCl, 1 mM MgCl 2 , 1 mM TCEP, 0.01% Tween 20 and 1 μM GppNHp, treated with 66 nM fluorescein-labelled peptides and incubated for 4 h at room temperature. Fluorescence polarization values ( λ ex =470 nm, λ em =525 nm) were determined at room temperature. Initial studies for alkyne macrocyclized peptides were performed as single measurements. Final affinity measurements of a subset of peptides were performed in triplicates. After correction for changes in fluorescence intensity upon binding, the fluorescence anisotoropy data were converted into fraction bound of the FITC-labelled peptide and fitted to a one-site binding model derived from the law of mass action using K d as the only fitting parameter (for details, see Supplementary Methods ) [63] . Nonlinear regression was performed in Prism 5.0 (Graphpad) [64] . Competition fluorescence polarization assay Acetylated peptides were serially diluted and incubated with a mixture of the fluorescein-labelled peptide and Rab8a 6–176 (GppNHp) at room temperature for 1 h. Fluorescence polarization was determined and IC 50 values were calculated by nonlinear regression analysis using Prism 5.0 software (GraphPad) [64] . How to cite this article: Cromm, P. M. et al . Orthogonal ring-closing alkyne and olefin metathesis for the synthesis of small GTPase-targeting bicyclic peptides. Nat. Commun. 7:11300 doi: 10.1038/ncomms11300 (2016).